Hot photocarrier dynamics in organic solar cells Photocurrent in an organic solar cell is generated by a charge transfer reaction between electron donors and acceptors. Charge transfer is expected to proceed from thermalized states, but this picture has been challenged by recent studies that have investigated the role of hot excitons. Here we show a direct link between excess excitation energy and photocarrier mobility. Charge transfer from excited donor molecules generates hot photocarriers with excess energy coming from the offset between the lowest unoccupied molecular orbital of the donor and that of the acceptor. Hot photocarriers manifest themselves through a short-lived spike in terahertz photoconductivity that decays on a picosecond timescale as carriers thermalize. Different dynamics are observed when exciting the acceptor at its absorption edge to a thermalized state. Charge transfer in this case generates thermalized carriers described by terahertz photoconductivity dynamics consisting of an instrument-limited rise to a long-lived signal. Organic solar cells show increasing promise for renewable energy [1] , [2] with rapid progress over the past decade leading to power conversion efficiencies >10% (refs 3 , 4 ). The greatest advances have come from improved control over sample morphology [5] , [6] and the development of novel electron donors [7] , [8] . As the performance of organic solar cells approaches the limits envisaged with fullerene acceptors [9] , development of new donor/acceptor systems requires a more thorough theoretical understanding of what drives the charge transfer reaction and experimental tools to probe these processes [10] . One pathway to new systems is to use excess excitation energy to drive the charge transfer reaction. Several recent studies have concluded that hot charge transfer states boost the charge generation yield [11] , [12] , [13] . Bakulin et al . [14] showed that delocalization could be induced by excited state absorption, which in turn led to a rise in photocurrent. While these studies examine excited state dynamics, optical pump-probe measurements cannot address the relationship between excess energy and carrier mobility. Time-resolved terahertz spectroscopy (TRTS) probes photoconductivity with the temporal resolution needed to access donor–acceptor interactions in real time [15] . TRTS yields valuable insight, but it is an open question whether the initial terahertz photoconductivity dynamics in organic semiconductors are due to carrier localization [15] , [16] or recombination [17] , [18] , [19] . Here we address these issues by combining TRTS with transient absorption (TA) spectroscopy and through selective excitation of the electron donor or acceptor. We show that the short-lived terahertz photoconductivity is the signature of a hot electron and its magnitude is sensitive to the interfacial volume between donors and acceptors. Efficient charge transfer is found when exciting the electron acceptor at its absorption edge, demonstrating that the excess energy of a hot photocarrier is not necessary to initiate the charge transfer reaction. Model system for charge transfer We selected three widely studied materials with technological relevance as model systems for charge transfer: buckminsterfullerene (C 60 ) is the electron acceptor and zinc phthalocyanine (ZnPc) and alpha-sexithiophene (α-6T) are the electron donors. Cnops et al . [20] achieved organic solar cells with a power conversion efficiency of 8.4% with using an α-6T donor and subphthalocyanine acceptors and the 12% record efficiency for organic solar cells was achieved in a sublimed tandem structure [3] . 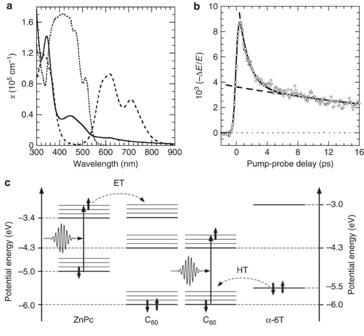Figure 1: Absorption spectra, a sample terahertz transient, and charge transfer processes. (a) Absorption spectra of C60(solid line), ZnPc (dashed line) and α-6T (dotted line). (b) Sample THz transient (circles) fit to double exponential decay (dashed lines) and error function rise time (solid line). (c) Illustration of electron transfer and hole transfer processes. Figure 1a shows the absorption spectra of C 60 , ZnPc and α-6T. Figure 1b shows an example of terahertz photoconductivity dynamics, measured by scanning the delay between optical pump and terahertz probe with the system set to sample the peak of the terahertz electric field E ( t ). The experimental data is fit to biexponential decay over the first 20 ps following excitation: Figure 1: Absorption spectra, a sample terahertz transient, and charge transfer processes. ( a ) Absorption spectra of C 60 (solid line), ZnPc (dashed line) and α-6T (dotted line). ( b ) Sample THz transient (circles) fit to double exponential decay (dashed lines) and error function rise time (solid line). ( c ) Illustration of electron transfer and hole transfer processes. Full size image The slower decay constant t 2 was determined by a linear regression where t / t 1 >>1 and then the residual was similarly fit. The rise in terahertz photoconductivity is well described by an error function with a rise time ( t 0 ) of ∼ 0.3 ps. TA [11] , [12] , [13] , [14] and broadband ( ∼ 10 THz) terahertz photoconductivity [15] studies have shown that charge transfer occurs within 0.1 ps, so we consider the rise to be instrument limited by the bandwidth of the spectrometer ( ∼ 3 THz). The decay dynamics of donor/acceptor films are complex, in part due to parallel charge transfer processes. These include charge transfer from an excited donor to an unoccupied orbital of the acceptor (electron transfer), charge transfer from an occupied orbital of the electron donor to an excited acceptor (hole transfer), as well as charge transfer between molecules of the same type (autoionization) [21] . We disentangle these processes, shown in Fig. 1c , by varying the sample composition and through selective excitation of the electron donor or acceptor. We focus on multi-layered structures as these enable us to vary the interfacial volume while maintaining the superior mobility of neat films. Alternate deposition of ultrathin layers yields a phase-segregated morphology with superior charge transport vis-à-vis co-sublimed blends [22] . Terahertz photoconductivity of films with C 60 and ZnPc We first consider terahertz photoconductivity following electron transfer from an excited donor molecule. 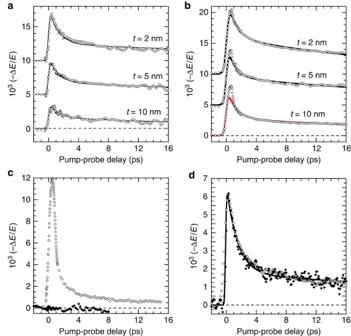Figure 2: Terahertz photoconductivity dynamics of films with C60and ZnPc. THz transients of layered films excited at (a) 615 nm and (b) 400 nm. Lines show fit to equation (1). (c) THz transients of neat C60, excited at 400 nm (open) or 615 nm (filled). (d) TRTS pump scans of 1:1 blends of C60and ZnPc, excited at 400 nm (open) or 615 nm (filled), normalized to the peak signal. Figure 2a shows pump scans of layered C 60 /ZnPc films excited at 615 nm and fits to the data. The fitting parameters of equation (1) are shown in Table 1 . The extinction coefficient of ZnPc (92,500 cm −1 ) is nine times that of C 60 (10,200 cm −1 ) at 615 nm such that ZnPc is preferentially excited. The signal magnitude increases as the layer thickness decreases, but the initial decay rate is independent of layer thickness. TA measurements of C 60 /ZnPc films show no significant recombination over the first 10 ps following charge transfer [19] . Hence, the early terahertz dynamics in the layered system arise from a reduction in mobility as transferred carriers thermalize and become localized. This interpretation is consistent with Cooke et al . [15] , who showed that charge carriers in polymer:fullerene blends localize within 1 ps. The initial terahertz photoconductivity dynamics observed for donor–acceptor systems, thus, arise from ultrafast charge transfer following excitation of a donor molecule at a heterojunction, followed by decay due to decreasing mobility as the carrier localizes. Excitation of a donor molecule within a layer, on the other hand, requires exciton migration to the interface before charge transfer. For the exciton diffusivity in organic semiconductors (10 −6 m 2 s −1 ) [23] , exciton diffusion to an interface requires ∼ 10 ps. Charge transfer from molecules excited within a layer does not contribute to the initial transient, which in turn decreases with increasing layer thickness. Figure 2: Terahertz photoconductivity dynamics of films with C 60 and ZnPc. THz transients of layered films excited at ( a ) 615 nm and ( b ) 400 nm. Lines show fit to equation (1). ( c ) THz transients of neat C 60 , excited at 400 nm (open) or 615 nm (filled). ( d ) TRTS pump scans of 1:1 blends of C 60 and ZnPc, excited at 400 nm (open) or 615 nm (filled), normalized to the peak signal. Full size image Table 1 Fitting parameters for the THz transients of layered C 60 /ZnPc and C 60 /α-6T films. Full size table Decay dynamics are more complex when both the donor and acceptor are excited. Figure 2b shows pump scans of layered C 60 /ZnPc films for excitation at 400 nm. Weaker trends in the peak signal magnitude are observed but the initial decay is sensitive to layer thickness. Using the same decay parameters as above, we obtained good fits for all dynamics for t >1 ps and a similar trend with increasing layer thickness. There is an additional short-lived component to the signal that increases in magnitude with increasing layer thickness. This component has the same dynamics as for excitation of neat C 60 at 400 nm ( Fig. 2c ). Excitation of C 60 molecules within a separate domain results in autoionization and recombination to a neutral exited state, contributing an additional short-lived component to the terahertz response of the film. No significant terahertz photoconductivity was observed following excitation of C 60 at 615 nm ( Fig. 2c ). The absorption edge of solid C 60 is at ∼ 750 nm and, thus, the excess energy ( ∼ 0.3 eV) is insufficient for autoionization. The presence of a neighbouring electron provides competing pathway to autoionization and, thus, there is little difference in dynamics when exciting at different wavelengths for films with the thinnest layers. This is most evident when comparing the terahertz photoconductivity dynamics of a 1:1 composite film, excited at 400 or 615 nm ( Fig. 2d ). The rise time is faster for excitation at 615 nm as with layered films, but the decay dynamics are not affected by the excitation wavelength. Transfer of an electron follows excitation of ZnPc at 400 or 615 nm to an upper excited state of C 60 , generating a hot carrier. Charge transfer also occurs following excitation of C 60 , a process analogous to hole transfer. In that case, C 60 is excited to a higher lying Franck–Condon level and charge transfer precedes thermalization. The excess excitation energy results in the same terahertz photoconductivity decay dynamics when the donor is excited. Terahertz photoconductivity of films with C 60 and α-6T Measurements of C 60 /α-6T films give further weight to our interpretation that the initial decay of terahertz photoconductivity arises from thermalization of a transferred photocarrier. The absorption spectra of C 60 and α-6T permit the selective excitation of either molecule as the extinction coefficient of α-6T (169,000 cm −1 ) is 4.8 times that of C 60 at 400 nm (35,000 cm −1 ), but α-6T does not absorb at 615 nm ( Fig. 1a ). 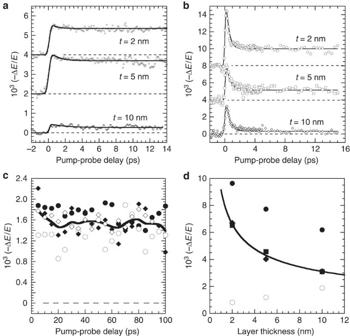Figure 3: Terahertz photoconductivity dynamics of films with C60and α-6T. THz transients of layered films of C60and α-6T, excited at (a) 615 nm or (b) 400 nm. (c) Zero to 100 ps delayed transients of 2 nm (circles) and 5 nm (diamonds) layered films of C60and α-6T, excited at 400 nm (filled symbols) and 615 nm (open symbols). The line shows an average of all data sets. (d) Dependence of the peak terahertz photoconductivity on layer thickness for C60/ZnPc films excited at 615 nm (squares), C60/α-6T films excited at 400 nm (diamonds) and C60/ZnPc films excited at 400 nm, broken down into the contributions from autoionization (open circles) and charge transfer (filled circles). Figure 3a shows the terahertz photoconductivity dynamics following excitation of the electron acceptor (C 60 at 615 nm) and Fig. 3b shows the terahertz photoconductivity dynamics following excitation of the electron donor (α-6T at 400 nm). When exciting the electron acceptor, there is a sharp rise ( t 0 =0.3 ps) to an equilibrium signal with only a weak overshoot ( ∼ 10% of the initial signal). The terahertz photoconductivity is stable out to a delay of 100 ps, shown in Fig. 3c . The terahertz photoconductivity dynamics arise from electron transfer from α-6T to an excited C 60 molecule. As the excitation is near the absorption edge, the resulting photocarrier is thermalized and hence there is no short-lived terahertz photoconductivity. This result demonstrates unambiguously that efficient charge transfer occurs from thermalized states. Even though the absorbance of C 60 /α-6T films is relatively weak at 615 nm ( ∼ 50% of incident radiation is absorbed), the magnitude of the long-lived signal is comparable to that following charge transfer with excess energy. Figure 3: Terahertz photoconductivity dynamics of films with C 60 and α-6T. THz transients of layered films of C 60 and α-6T, excited at ( a ) 615 nm or ( b ) 400 nm. ( c ) Zero to 100 ps delayed transients of 2 nm (circles) and 5 nm (diamonds) layered films of C 60 and α-6T, excited at 400 nm (filled symbols) and 615 nm (open symbols). The line shows an average of all data sets. ( d ) Dependence of the peak terahertz photoconductivity on layer thickness for C 60 /ZnPc films excited at 615 nm (squares), C 60 /α-6T films excited at 400 nm (diamonds) and C 60 /ZnPc films excited at 400 nm, broken down into the contributions from autoionization (open circles) and charge transfer (filled circles). Full size image When exciting the electron donor α-6T at 400 nm, however, the terahertz photoconductivity dynamics ( Fig. 3b ) are qualitatively similar to those measured following excitation of ZnPc—a short-lived transient, followed by a long-lived component. The decay dynamics are significantly faster for C 60 /α-6T than for C 60 /ZnPc (see Table 1 ) with the equilibrium value being reached within 2 ps. The faster decay dynamics may reflect differences in transfer dynamics as the hot carrier is transferred to C 60 in both cases. As with excitation of C 60 /α-6T at 615 nm, the terahertz photoconductivity is stable up to 100 ps delay. There is a remarkable agreement between the magnitude of the initial peak in terahertz photoconductivity when exciting the donor, shown in Fig. 3d . For both C 60 /ZnPc and C 60 /α-6T films, the signal scales inversely with the square root of layer thickness (solid line). The absorbance of the two films at the pump wavelength is similar (>97%) and the same photon flux was used. As the hole mobility of polycrystalline α-6T films (ca. 10 −2 cm 2 V −1 s) [24] is two orders of magnitude larger than that of ZnPc (ca. 10 −4 cm 2 V −1 s) [25] , the initial photoconductivity dynamics following electron transfer from an excited donor molecule reflect thermalization of the transferred carrier rather than relaxation of the electron donor. The same trend is seen for excitation of C 60 /ZnPc films at 400 nm after neglecting the contribution from autoionization. The signal is higher, reflecting the additional contribution of hole transfer following excitation of C 60 . Finally, the autoionization transient increases with layer thickness as an increasing fraction of excited C 60 molecules lie within a separate domain. Transient absorption of films with C 60 and α-6T Regardless as to whether the donor or acceptor is excited, the terahertz photoconductivity of C 60 /α-6T films is stable from ∼ 5 to 100 ps pump-probe delay. We performed TA measurements to correlate TRTS with excited state populations. 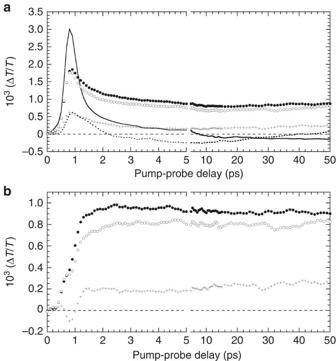Figure 4: Transient absorption dynamics of films with C60and α-6T. (a) Transient absorption dynamics of C60(solid line), α-6T (dashed line) and layered films with 2 nm (filled circles), 5 nm (open circles) and 10 nm (crosses) thick layers, probed at 470 nm. (b) Change in the transient absorption dynamics of layered films relative to neat films. Figure 4a shows the TA of C 60 , α-6T and layered films excited at 387.5 nm and probed at 470 nm. The probe wavelength was selected where there are minimal contributions from α-6T and C 60 (see Supplementary Fig. 1 ) and, thus, absorption bleaching dynamics can be tracked with minimal interference. Neat films show a short-lived transient bleaching (decay constants 0.5 ps for C 60 ; 1.1 ps for α-6T) with a crossover to TA at 6 ps for C 60 and 2 ps for α-6T. The correlation between the TA and THz decay dynamics (see Fig. 2 ) led us to assign the short-lived state in C 60 to autoioinization. Lanzani et al . [26] previously identified a short-lived intrachain singlet state of α-6T that converts to a charge transfer state within several picoseconds. The layered films have a short-lived component similar to that of α-6T, but exhibit long-lived bleaching of ground-state absorption that increases with decreasing layer thickness. The initial dynamics reflect a combination of transient bleaching and absorption of neutral as well as charged states. We eliminated the contribution of neutral states to the transient transmission dynamics by subtracting off a scaled fraction of the neat film to eliminate the initial decay ( Fig. 4b ). The resulting dynamics match the terahertz photoconductivity and scale similarly with layer thickness. Figure 4: Transient absorption dynamics of films with C 60 and α-6T. ( a ) Transient absorption dynamics of C 60 (solid line), α-6T (dashed line) and layered films with 2 nm (filled circles), 5 nm (open circles) and 10 nm (crosses) thick layers, probed at 470 nm. ( b ) Change in the transient absorption dynamics of layered films relative to neat films. Full size image In summary, we find that charge transfer to a state with excess energy generates a hot photocarrier that localizes within a picosecond. Photogeneration of a hot carrier manifests itself through short-lived terahertz photoconductivity that decays on a picosecond timescale. The insensitivity of the photoconductivity magnitude to hole mobility suggests that C 60 anions are the dominant contributor to terahertz photoconductivity in the films studied here. Excitation of the electron acceptor at its optical gap generates localized photocarriers, demonstrating efficient charge transfer even in the absence of excess excitation energy. These results illustrate the value of terahertz spectroscopy for probing charge transfer reactions at organic heterojunctions. Sample preparation C 60 , α-6T and ZnPc were purified by consecutive vacuum train sublimation before use. We did not use a functionalized fullerene such as phenyl-C61-butyric acid methyl ester (PCBM), because such materials partially decompose under sublimation. Films ( ∼ 300 nm thick) were prepared by sublimation under dynamic vacuum (3.0 × 10 −7 Torr) from resistive heating furnaces onto fused silica substrates that were cleaned with organic solvents and subjected to ozone treatment prior to use. Films with a layered nanostructure were prepared by alternate layer deposition and composite films were prepared by co-sublimation. Quartz crystal microbalances were used to monitor the rate of deposition and determine the film composition and layer thickness. The absorption spectra of the films were measured using a spectrophotometer (Lambda 1,050, Perkin Elmer). A custom spectrometer with an integrating sphere was used to measure absorption at low absorbance levels. Terahertz spectroscopy The terahertz spectrometer is driven by 60 fs pulses from a kilohertz Ti:Sapphire amplifier and interrogated with optically gated and synchronized terahertz probe pulses. The output of the amplifier passed through a 50/50 beam splitter and the resulting pulses were used to generate the terahertz probe and optical pump pulses. Probe pulses were generated by a 2-mm thick ZnTe[110] crystal and detected using a matched ZnTe crystal and free-space electro-optical sampling. The output of the Ti:sapphire amplifier was frequency doubled by a β-BaB 2 O 4 crystal to 400 nm or used to excite a near infrared optical parametric amplifier and then frequency doubled to 615 nm. The pump intensity was 20 μJ per pulse at 615 nm or 30 μJ per pulse at 400 nm (6 × 10 13 photons per cm 2 per pulse). All measurements were performed in the linear regime for this spectrometer (see Supplementary Fig. 2 ). The temporal dynamics of the terahertz photoconductivity were measured by scanning the delay between the pump and probe beam with the probe gated such that the peak of the terahertz pulse was sampled. There is a slight phase shift between the peak of the terahertz pulse and the change in the terahertz transmission, although the amplitude does not change significantly (see Supplementary Fig. 3 ). The peak of the pump-induced change in terahertz transmission was not affected by changing the pump-probe delay. Transient absorption TA experiments were based on a 1 kHz Ti:Sapphire amplifier (775 nm). A portion of the output was frequency doubled by a β-BaB 2 O 4 crystal for sample excitation. A small amount of power was focused into a sapphire plate to produce the white-light continuum probe. The excited state spectra were resolved using a scanning monochromator. Ground-state bleach and excited state absorption dynamics were recorded by adjusting the delay between the pump and probe pulses. The pump fluence was adjusted to ∼ 6 × 10 13 photons per cm 2 per pulse. A temporal resolution of ∼ 280 fs was measured through cross-correlation. How to cite this article: Lane, P. A. et al . Hot photocarrier dynamics in organic solar cells. Nat. Commun. 6:7558 doi: 10.1038/ncomms8558 (2015).